Lin28/let-7 axis regulates aerobic glycolysis and cancer progression via PDK1 Aberrant expression of Lin28 and let-7 has been observed in many human malignancies. However, its functions and underlying mechanisms remain largely elusive. Here we show that aberrant expression of Lin28 and let-7 facilitates aerobic glycolysis, or Warburg effect, in cancer cells. Mechanistically, we discover that Lin28A and Lin28B enhance, whereas let-7 suppresses, aerobic glycolysis via targeting pyruvate dehydrogenase kinase 1, or PDK1, in a hypoxia- or hypoxia-inducible factor-1 (HIF-1)-independent manner, illustrating a novel pathway to mediate aerobic glycolysis of cancer cells even in ambient oxygen levels. Importantly, we further demonstrate that PDK1 is critical for Lin28A- and Lin28B-mediated cancer proliferation both in vitro and in vivo , establishing a previously unappreciated mechanism by which Lin28/let-7 axis facilitates Warburg effect to promote cancer progression. Our findings suggest a potential rationale to target PDK1 for cancer therapy in malignancies with aberrant expression of Lin28 and let-7. A recognized hallmark of cancer is aerobic glycolysis or the Warburg effect, which is a phenomenon described by Warburg over 90 years ago that cancer cells rely heavily on glycolytic fermentation for energy metabolism even with ambient oxygen supply [1] . While the Warburg effect is now well appreciated [2] , the mechanisms driving aerobic glycolysis are not fully understood. As cancer evolves by many different mechanisms that confer cancer cells with various abilities or hallmarks that distinguish cancer cells from their normal counterparts, researchers often ponder how and why cancer cells adapt to the less efficient aerobic glycolysis for energy metabolism. There is no doubt that cancer-specific metabolism is largely responsible for growth advantage of cancer cells and, therefore, deciphering mechanisms underlying aerobic glycolysis in cancer cells could potentially lead to new therapy of human malignancies [3] . A recent study reported that, in mouse diabetic models, Lin28A and Lin28B regulate glucose metabolism in vivo through modulating insulin-phosphoinositide 3-kinase-mammalian target of rapamycin (insulin-PI3K-mTOR) signalling via the let-7 microRNAs (miRNAs) [4] . This discovery may have significant relevance to understanding mechanisms for oncogenesis, considering the fact that aberrant expression of Lin28 and let-7 has been observed in 10–20% of human cancers [5] , [6] , [7] . The RNA-binding protein Lin28A and its homologue Lin28B are known to play key roles in cell growth, germ lineage and are implicated in a variety of pathological states including cancer, obesity and diabetes [8] , [9] . In addition, they function as reprogramming factors, together with Oct4, Nanog and Sox2, to regulate the pluripotency of stem cells [10] . Lin28A and Lin28B control gene regulatory networks through multiple mechanisms, the best-studied being the regulation of Lin28 on let-7, one of the first miRNAs discovered in Caenorhabditis elegans , where Lin28 and let-7 have opposite effects on the developmental progression [11] , [12] , [13] , [14] . The Lin28/let-7 axis has been involved in cancer development in various ways. For instance, Lin28B expression was recently reported to promote the development of neuroblastomas through low let-7 miRNA levels and high MYCN protein expression [15] . In regard to metabolism regulation, besides above-mentioned regulatory roles of Lin28/let-7 axis on glucose metabolism in mouse diabetic models [4] , modulation of metabolic gene expression by Lin28 was also discovered by genome-wide study of human embryonic stem cells (ESC) [16] . Also in mouse ESC, Shyh-Chang et al. [17] documented that Lin28 and let-7 regulate threonine and S-adenosyl-methionine metabolism. More recently, Shyh-Chang et al. [18] reported that Lin28A bound to and enhanced the translation of mRNAs for several metabolic enzymes, thereby increasing not only glycolysis but also oxidative phosphorylation (OXPHOS) during tissue repair. Nevertheless, it is worthwhile to note that regulation of this axis on cancer cell metabolism has never been directly tested, at least to the best of our knowledge. Mounting evidence suggests that oncogenic alterations actively reprogram metabolism in cancer cells. For instance, proto-oncogene c-Myc , whose deregulation has been documented in ~30–50% human malignancies, is known to regulate many enzymes that facilitate glycolytic metabolism in cancer cells [19] . Another important oncogenic protein hypoxia-inducible factor-1 (HIF-1), whose activation caused by von Hippel–Lindau tumour suppressor mutation has been responsible for 90% of human renal carcinomas, is also known as a master regulator for cancer cell metabolism [20] , [21] , [22] . Zhang et al. [23] reported that HIF-1 promotes Warburg effect in renal cancer cells by negatively regulating mitochondrial biogenesis and O 2 consumption. Most notably, it is reported that HIF-1, via its direct target pyruvate dehydrogenase kinase 1 (PDK1), negatively regulates pyruvate dehydrogenase (PDH), thereby shutting down pyruvate entry into the tricarboxylic acid cycle (TCA) under hypoxic condition [24] , [25] . While those studies elegantly illustrated metabolic switch under hypoxic condition, they could not explain sufficiently why cancer cells adapt aerobic glycolysis, that is, cancer cells rely heavily on the wasteful glycolysis for energy supply, even under oxygen rich conditions. Therefore, a provocative question remains to be answered to understand more adequately the central dogma of Warburg effect: what is the molecular basis that facilitates metabolic switch in cancer cells under normal oxygen conditions? It is recognized that both transcriptional and post-transcriptional mechanisms are involved in regulating cancer metabolism [2] , [26] . However, compared with accumulating documentations of genetic alterations and their transcriptional regulation of metabolic pathways in cancer cells, little is known about post-transcriptional miRNA-mediated regulation of cancer metabolism. In the present study, we seek to determine whether and how aberrant expression of Lin28 and let-7 could reprogram cancer metabolism. We demonstrate that Lin28A and Lin28B enhance, whereas let-7 suppresses, aerobic glycolysis in cancer cells. We discover that Lin28/let-7 axis regulates cancer cell metabolism by targeting PDK1 in a hypoxia- or HIF-1-independent manner. Importantly, we further demonstrate that PDK1 expression is critical for Lin28A- and Lin28B-mediated cancer proliferation both in vitro and in vivo . Thus, our results establish a previously unappreciated mechanism by which Lin28/let-7 axis facilitates Warburg effect and cancer progression. Aberrant expression of Lin28A/B and let-7g in cancer cells Previous studies have documented that Lin28A, Lin28B and let-7 were aberrantly expressed in human malignancies [6] . In this study, we analysed 17 pairs of human hepatocellular carcinoma (HCC) lesions and corresponding normal adjacent tissues with real-time PCR and observed that Lin28A and Lin28B had higher expression in HCC samples compared with normal adjacent tissues ( Fig. 1a,b and Supplementary Fig. 1A,B ). In contrast, let-7g expression was decreased in HCC samples compared with normal adjacent tissues ( Fig. 1c and Supplementary Fig. 1C ). Western blot analysis demonstrated high expression of both Lin28A and Lin28B in several cancer cell lines, including Hep3B, one of HCC cell lines ( Fig. 1d ). To further determine the physiological relevance of high expression of Lin28A and Lin28B in cancer cells, we established Hep3B cells stably expressing short hairpin RNAs (shRNAs) targeting Lin28A or Lin28B, and found that downregulation of Lin28A or Lin28B by shRNAs significantly impaired the proliferation of Hep3B cells ( Fig. 1e and Supplementary Fig. 2A,B ). We also detected their effect on the proliferation with siRNAs targeting Lin28A and Lin28B. The results showed that Lin28A or Lin28B knockdown by siRNAs significantly inhibited the proliferation of Hep3B, which is consistent with shRNAs results, indicating a pro-proliferative effect of Lin28 in cancer cells ( Supplementary Fig. 2C,D ). On the other hand, let-7g mimics significantly suppressed the proliferation of Hep3B cells ( Fig. 1f ). Thus, these data demonstrated that Lin28A, Lin28B and let-7 were aberrantly expressed in HCC lesions and human cancer cell lines, indicating that this axis may play important roles in human cancer development. 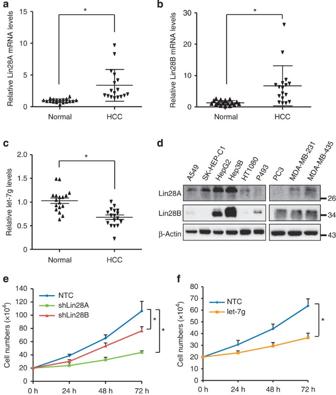Figure 1: Aberrant expression of Lin28A/B and let-7 g in cancer cells. (a–c) Lin28A, Lin28B and let-7g expression were determined by real-time qPCR in human HCC samples, values are given as the mean (±s.d.).n=17 in each group. *P<0.05 as compared with normal control group. (Student’st-test). (d) Protein levels of Lin28A and Lin28B were determined by western blot in different cancer cells. β-Actin served as loading control. (e,f) Cell growth of Hep3B cells stably expressing non-targeting control (NTC), shLin28A, shLin28B (e) or Hep3B cells transfected with NTC or let-7g mimics (f) were determined by Trypan blue staining. Data were presented as mean (±s.d.).n=3 in each group. *P<0.05 as compared with NTC control group (Student’st-test). Figure 1: Aberrant expression of Lin28A/B and let-7 g in cancer cells. ( a – c ) Lin28A, Lin28B and let-7g expression were determined by real-time qPCR in human HCC samples, values are given as the mean (±s.d.). n =17 in each group. * P <0.05 as compared with normal control group. (Student’s t -test). ( d ) Protein levels of Lin28A and Lin28B were determined by western blot in different cancer cells. β-Actin served as loading control. ( e , f ) Cell growth of Hep3B cells stably expressing non-targeting control (NTC), shLin28A, shLin28B ( e ) or Hep3B cells transfected with NTC or let-7g mimics ( f ) were determined by Trypan blue staining. Data were presented as mean (±s.d.). n =3 in each group. * P <0.05 as compared with NTC control group (Student’s t -test). Full size image Lin28A/B promote Warburg effect in cancer cells Recently, Lin28A and Lin28B were found to regulate glucose metabolism in mouse diabetic models to improve glucose tolerance [4] . We hypothesized that aberrant expression of Lin28A and Lin28B in cancer cells could also regulate aerobic glycolysis, one of the hallmarks of cancer, to facilitate cancer proliferation. To test this hypothesis, we established Hep3B cells stably expressing Lin28A or Lin28B using virus infection followed by puromycin selection ( Fig. 2a ). Measurement of metabolic parameters revealed that cellular glucose uptake and lactate production in culture medium were increased significantly in Hep3B cells overexpressing either Lin28A or Lin28B ( Fig. 2b,c ). Moreover, forced expression of Lin28A or Lin28B led to increased cellular ATP levels and reduced cellular O 2 consumption rates ( Fig. 2d,e ). Similar results were observed in HT1080 cells ( Supplementary Fig. 3 ), SK-HEP-1 cells and PC3 cells ( Supplementary Fig. 4 ) stably overexpressing Lin28A or Lin28B. 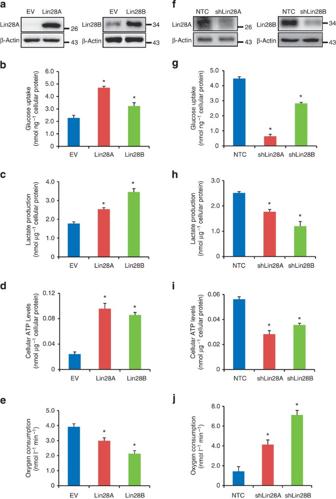Figure 2: Lin28A/B promote Warburg effect in cancer cells. (a) Lin28A and Lin28B protein levels were determined by western blot in Hep3B cells stably overexpressing empty vector (EV), Lin28A or Lin28B. β-Actin served as loading control. (b–e) Glucose uptake (b), lactate production (c), cellular ATP levels (d) and O2consumption (e) were measured in Hep3B cells stably overexpressing EV, Lin28A or Lin28B. Data were presented as mean (±s.d.).n=3 in each group. *P<0.05 as compared with EV group. (Student’st-test). (f) Lin28A and Lin28B protein levels were determined by western blot in Hep3B cells stably expressing non-targeting control (NTC), shLin28A or shLin28B. β-Actin served as loading control. (g–j) Glucose uptake (g), lactate production (h), cellular ATP levels (i) and O2consumption (j) were measured in Hep3B cells stably expressing NTC, shLin28A or shLin28B. Data were presented as mean (±s.d.).n=3 in each group. *P<0.05 as compared with NTC group. (Student’st-test). Figure 2: Lin28A/B promote Warburg effect in cancer cells. ( a ) Lin28A and Lin28B protein levels were determined by western blot in Hep3B cells stably overexpressing empty vector (EV), Lin28A or Lin28B. β-Actin served as loading control. ( b – e ) Glucose uptake ( b ), lactate production ( c ), cellular ATP levels ( d ) and O 2 consumption ( e ) were measured in Hep3B cells stably overexpressing EV, Lin28A or Lin28B. Data were presented as mean (±s.d.). n =3 in each group. * P <0.05 as compared with EV group. (Student’s t -test). ( f ) Lin28A and Lin28B protein levels were determined by western blot in Hep3B cells stably expressing non-targeting control (NTC), shLin28A or shLin28B. β-Actin served as loading control. ( g – j ) Glucose uptake ( g ), lactate production ( h ), cellular ATP levels ( i ) and O 2 consumption ( j ) were measured in Hep3B cells stably expressing NTC, shLin28A or shLin28B. Data were presented as mean (±s.d.). n =3 in each group. * P <0.05 as compared with NTC group. (Student’s t -test). Full size image In complementary loss-of-function studies, Hep3B cells stably expressing shRNAs targeting Lin28A or Lin28B were used ( Fig. 2f ). Cellular glucose uptake, lactate levels in medium and cellular ATP production were significantly decreased ( Fig. 2g–i ), whereas O 2 consumption rate was markedly increased ( Fig. 2j ), in Hep3B cells expressing shLin28A or shLin28B. Thus, our results from both gain-of-function and loss-of-function studies led to the conclusion that both Lin28A and Lin28B facilitated aerobic glycolysis, or Warburg effect, in cancer cells. Let-7 suppresses Warburg effect in cancer cells Let-7 family miRNAs have been reported to be blocked for maturation by both Lin28A and Lin28B (ref. 27 ). In this study, we also observed that overexpression of Lin28A or Lin28B markedly inhibited the expression of mature let-7 family miRNAs in Hep3B cells ( Supplementary Fig. 5A,B ). To determine whether miRNAs of let-7 family regulate cancer cell metabolism, we transfected Hep3B cells with miRNA mimics of let-7a, -7c, -7d, -7g or -7f. Opposite to the effect of Lin28A and Lin28B, most of the miRNAs of let-7 family reduced both cellular glucose uptake and lactate production in Hep3B cells ( Supplementary Fig. 5C,D ), with let-7g being the most efficient one. Of note, using the same HCC samples, we analysed two other let-7 species. The results indicated that let-7a and let-7c were also suppressed to a different degree compared with adjacent normal tissues ( Supplementary Fig. 6 ). However, let-7g is still the most widely altered compared with other let-7 species ( Supplementary Fig. 1C ). Hence, we next focused on let-7g to investigate its roles in aerobic glycolysis in cancer cells. Forced expression of let-7g ( Fig. 3a ) significantly reduced glucose uptake, lactate production and ATP levels ( Fig. 3b–d ), while markedly increased O 2 consumption compared with the non-targeting control (NTC) group ( Fig. 3e ). Similar results were obtained in HT1080 cells expressing let-7g mimics ( Supplementary Fig. 5E–G ). On the other hand, inhibition of let-7g by antagomirs ( Fig. 3f ) led to enhanced glucose uptake, lactate production and ATP levels in Hep3B cells ( Fig. 3g–i ). Taken together, these data suggested that let-7 family miRNAs, most notably let-7g, repressed aerobic glycolysis, or Warburg effect, in human cancer cells. 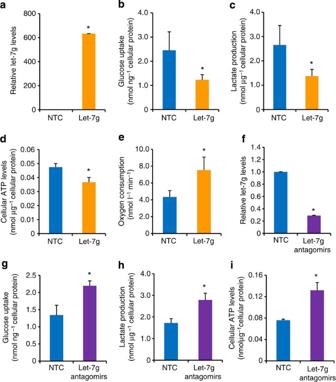Figure 3: Let-7g suppresses Warburg effect in cancer cells. (a) RT–qPCR analysis of let-7g expression in Hep3B cells transfected with NTC or let-7g mimics. Data were presented as mean (±s.d.).n=3 in each group. *P<0.05 as compared with NTC group (Student’st-test). (b–e) Glucose uptake (b), lactate production (c), ATP levels (d) and O2consumption (e) were measured in Hep3B cells transfected with NTC or let-7g mimics. Data were presented as mean (±s.d.).n=3 in each group. *P<0.05 as compared with NTC group (Student’st-test). (f) RT–qPCR analysis of let-7g expression in Hep3B cells transfected with NTC or let-7g antagomirs. Data were presented as mean (±s.d.).n=3 in each group. *P<0.05 as compared with NTC group. (Student’st-test). (g–i) Glucose uptake (g), lactate production (h) and ATP levels (i) were measured in Hep3B cells transfected with NTC or let-7g antagomirs. Data were presented as mean (±s.d.).n=3 in each group. *P<0.05 as compared with NTC group. (Student’st-test). Figure 3: Let-7g suppresses Warburg effect in cancer cells. ( a ) RT–qPCR analysis of let-7g expression in Hep3B cells transfected with NTC or let-7g mimics. Data were presented as mean (±s.d.). n =3 in each group. * P <0.05 as compared with NTC group (Student’s t -test). ( b – e ) Glucose uptake ( b ), lactate production ( c ), ATP levels ( d ) and O 2 consumption ( e ) were measured in Hep3B cells transfected with NTC or let-7g mimics. Data were presented as mean (±s.d.). n =3 in each group. * P <0.05 as compared with NTC group (Student’s t -test). ( f ) RT–qPCR analysis of let-7g expression in Hep3B cells transfected with NTC or let-7g antagomirs. Data were presented as mean (±s.d.). n =3 in each group. * P <0.05 as compared with NTC group. (Student’s t -test). ( g – i ) Glucose uptake ( g ), lactate production ( h ) and ATP levels ( i ) were measured in Hep3B cells transfected with NTC or let-7g antagomirs. Data were presented as mean (±s.d.). n =3 in each group. * P <0.05 as compared with NTC group. (Student’s t -test). Full size image Lin28A/B regulate aerobic glycolysis via PDK1 Given that Lin28A and Lin28B regulate let-7 miRNAs in tumour cells, we asked whether Lin28A and Lin28B promote Warburg effect through upregulating let-7 target genes that are associated with glycolysis. Previous study by Zhu et al. [4] showed that Lin28/let-7 axis regulates glucose metabolism via targeting the insulin-Akt-mTOR pathway. However, when we examined the activation status of the Akt-mTOR pathway in Hep3B or HT1080 cells with different expression levels of Lin28A, Lin28B or let-7g, we observed that this pathway was only marginally affected by the Lin28/let-7 axis, as indicated by AKT and RPS6 phosphorylation levels ( Supplementary Fig. 7 ). We therefore concluded that other mechanisms might be involved in Lin28/let-7-mediated aerobic glycolysis in cancer cells. We then detected the protein expression of important enzymes involved in glucose metabolism in Hep3B cells overexpressing Lin28A or Lin28B. Interestingly, western blot analysis revealed that overexpression of Lin28A or Lin28B resulted in an obvious increase in PDK1 protein expression in Hep3B cells ( Fig. 4a ). Similar results were observed in HT1080, SK-HEP-1 and PC3 cells stably overexpressing Lin28A or Lin28B ( Supplementary Figs 4A,F and 9A ). However, neither Lin28A nor Lin28B affected PDK1 mRNA levels ( Supplementary Fig. 9B ), suggesting that PDK1 was regulated by Lin28A or Lin28B at post-transcriptional level. Consistently, downregulation of Lin28A or Lin28B by shRNAs reduced PDK1 protein levels in Hep3B cells ( Fig. 4b ). Of note, we also measured several important enzymes involved in the OXPHOS pathway, such as succinate dehydrogenase complex, subunit A (SDHA), PDH E1 component subunit alpha (PDHA1), citrate synthase (CS), isocitrate dehydrogenase 2 (IDH2) and fumarate hydratase (FH) in Hep3B cells stably overexpressing Lin28A or Lin28B, and the results displayed no obvious changes of these enzymes ( Fig. 4a and Supplementary Fig. 8A,B ). Of glycolysis enzymes, besides PDK1, triose-phosphate isomerase (TPI) was also mildly affected by Lin28A and Lin28B ( Fig. 4a ). 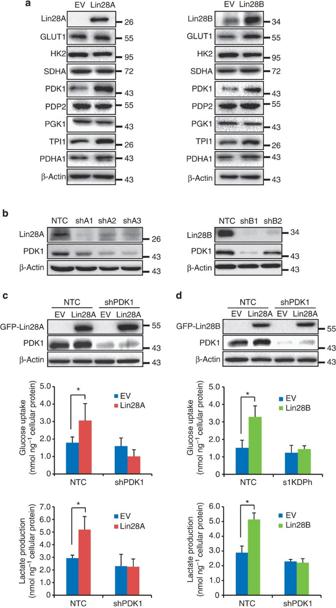Figure 4: Lin28A/B regulate aerobic glycolysis via PDK1. (a) Protein levels of metabolic enzymes were determined by western blot in Hep3B cells overexpressing empty vector (EV), Lin28A or Lin28B. β-Actin served as loading control. (b) PDK1 protein levels were measured by western blot in Hep3B cells stably expressing NTC, shLin28A or shLin28B. β-Actin served as loading control. (c) Hep3B cells stably overexpressing EV or GFP-Lin28A were further infected with viruses expressing NTC or shPDK1. PDK1 protein levels, cellular glucose uptake and lactate production in the medium were determined. Data were presented as mean (±s.d.).n=3 in each group. *P<0.05 as compared with indicated group. (Student’st-test). (d) Hep3B cells stably overexpressing EV or GFP-Lin28B were further infected with viruses expressing NTC or shPDK1. PDK1 protein levels, cellular glucose uptake and lactate production in the medium were determined. Data were presented as mean (±s.d.).n=3 in each group. *P<0.05 as compared with indicated group. (Student’st-test). Figure 4: Lin28A/B regulate aerobic glycolysis via PDK1. ( a ) Protein levels of metabolic enzymes were determined by western blot in Hep3B cells overexpressing empty vector (EV), Lin28A or Lin28B. β-Actin served as loading control. ( b ) PDK1 protein levels were measured by western blot in Hep3B cells stably expressing NTC, shLin28A or shLin28B. β-Actin served as loading control. ( c ) Hep3B cells stably overexpressing EV or GFP-Lin28A were further infected with viruses expressing NTC or shPDK1. PDK1 protein levels, cellular glucose uptake and lactate production in the medium were determined. Data were presented as mean (±s.d.). n =3 in each group. * P <0.05 as compared with indicated group. (Student’s t -test). ( d ) Hep3B cells stably overexpressing EV or GFP-Lin28B were further infected with viruses expressing NTC or shPDK1. PDK1 protein levels, cellular glucose uptake and lactate production in the medium were determined. Data were presented as mean (±s.d.). n =3 in each group. * P <0.05 as compared with indicated group. (Student’s t -test). Full size image Since PDK1 is a critical enzyme regulating glycolytic metabolism in cancer cells, we next sought to determine whether PDK1 is involved in elevated glycolysis regulated by Lin28A and Lin28B. We found that when PDK1 was knocked down by shRNAs in Hep3B cells, Lin28A- or Lin28B-induced increase in glucose uptake and lactate production was obviously attenuated ( Fig. 4c,d ), indicating that PDK1 is a functional downstream target of Lin28A and Lin28B to regulate aerobic glycolysis. PDK1 is known to facilitate metabolic switch in cancer cells by inactivating the TCA enzyme PDH that converts pyruvate to acetyl-CoA [24] , [28] . To confirm that Lin28A and Lin28B decreased OXPHOS process, we measured PDH activity in Hep3B using a PDH activity assay kit. The results showed that cellular PDH activity decreased significantly in Hep3B cells overexpressing either Lin28A or Lin28B ( Supplementary Fig. 10A ). While forced expression of siLin28A or siLin28B led to increased PDH activity ( Supplementary Fig. 10B ). Collectively, these data suggest that Lin28A and Lin28B promote glycolysis while inhibiting OXPHOS process. PDK1 is a direct target of Let-7g Next, we analysed the expression of metabolic enzymes in Hep3B cells transfected with let-7g mimics. Our results revealed that let-7g mimics significantly suppressed PDK1 protein expression in Hep3B cells ( Fig. 5a ), with no obvious effects on other enzymes, specifically those important OXPHOS enzymes, such as SDHA, PDHA1, CS, IDH2 and FH ( Fig. 5a and Supplementary Fig. 8C ), suggesting that PDK1 might be a target gene of let-7g. Contrast to decreased PDK1 protein expression by let-7g mimics, let-7g antagomirs increased PDK1 protein expression in both Hep3B and HT1080 cells ( Fig. 5b ). Similar results were observed in PLC, HepG2 and P493 cells expressing let-7g mimics ( Supplementary Fig. 11 ). Further experiments showed that let-7g had no effect on PDK1 mRNA levels ( Fig. 5c ), indicating that PDK1 was regulated by let-7g at post-transcriptional level. Moreover, forced expression of let-7g mimics markedly increased the PDH activity and inhibition of let-7g by antagomirs led to reduced PDH activity ( Supplementary Fig. 10C,D ), suggesting that let-7g regulates glycolysis via PDK1 inactivation. 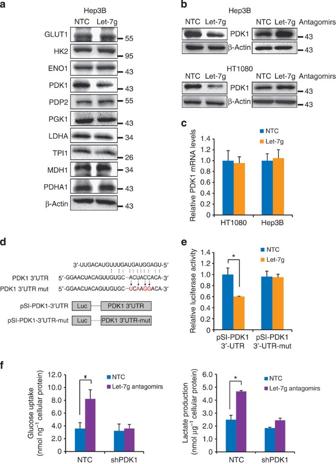Figure 5: PDK1 is a direct target of let-7g. (a) Protein levels of metabolic enzymes were determined by western blot in Hep3B cells expressing NTC or let-7g mimics. β-Actin served as loading control. (b) PDK1 protein levels were determined by western blot in Hep3B and HT1080 cells expressing NTC or let-7g mimics or let-7g antagomirs. β-Actin served as loading control. (c) PDK1 mRNA levels were measured by RT–qPCR in HT1080 and Hep3B cells expressing NTC or let-7g mimics. Data were presented as mean (±s.d.).n=3 in each group. (d) Predicted base pairing between let-7g and 3′UTR ofPDK1by RNAhybrid software. Wild-type or mutated (mut) 3′UTR of PDK1 sequence inserted into dual-luciferase vector were shown. (e) Let-7g mimics were co-transfected withpSI-PDK1-3′UTRorpSI-PDK1-3′UTR-mutinto HEK293 cells followed by dual-luciferase analysis. Data were presented as mean (±s.d.).n=3 in each group. *P<0.05 as compared with indicated group. (Student’st-test). (f) NTC or let-7g antagomirs were transfected into Hep3B cells stably expressing NTC or shPDK1, followed by measurement of cellular glucose uptake and lactate production in culture medium. Data were presented as mean (±s.d.).n=3 in each group. *P<0.05 as compared with indicated group (Student’st-test). Figure 5: PDK1 is a direct target of let-7g. ( a ) Protein levels of metabolic enzymes were determined by western blot in Hep3B cells expressing NTC or let-7g mimics. β-Actin served as loading control. ( b ) PDK1 protein levels were determined by western blot in Hep3B and HT1080 cells expressing NTC or let-7g mimics or let-7g antagomirs. β-Actin served as loading control. ( c ) PDK1 mRNA levels were measured by RT–qPCR in HT1080 and Hep3B cells expressing NTC or let-7g mimics. Data were presented as mean (±s.d.). n =3 in each group. ( d ) Predicted base pairing between let-7g and 3′UTR of PDK1 by RNAhybrid software. Wild-type or mutated (mut) 3′UTR of PDK1 sequence inserted into dual-luciferase vector were shown. ( e ) Let-7g mimics were co-transfected with pSI-PDK1-3′UTR or pSI-PDK1-3′UTR-mut into HEK293 cells followed by dual-luciferase analysis. Data were presented as mean (±s.d.). n =3 in each group. * P <0.05 as compared with indicated group. (Student’s t -test). ( f ) NTC or let-7g antagomirs were transfected into Hep3B cells stably expressing NTC or shPDK1, followed by measurement of cellular glucose uptake and lactate production in culture medium. Data were presented as mean (±s.d.). n =3 in each group. * P <0.05 as compared with indicated group (Student’s t -test). Full size image Bioinformatic analysis revealed that there is a potential let-7g binding fragment in the 3′-untranslated region (UTR) of PDK1 gene. We then cloned that potential let-7g binding fragment as well as its mutated form into a luciferase expressing pSI reporter vector ( Fig. 5d ). We found that forced expression of let-7g significantly suppressed the activity of the luciferase reporter gene containing the wild-type 3′UTR of PDK1 but not the one containing the mutated form ( Fig. 5e ), indicating that PDK1 is a direct target of let-7g. Next, we sought to examine whether PDK1 was involved in decreased glycolytic metabolism regulated by let-7g. We found that when PDK1 was stably knocked down by shRNAs in Hep3B cells, the effect of let-7g antagomirs on glucose uptake and lactate production was markedly attenuated ( Fig. 5f ), establishing PDK1 as a functional downstream target of let-7g in regulation of glycolytic metabolism. Lin28-regulated cancer cell metabolism is HIF-1-independent It has been shown that HIF-1 plays key roles in regulating glycolysis under hypoxic condition through activation of PDK1 (refs 24 , 25 ). However, given that the basal HIF-1 protein level is very low under normoxia, it is still a mystery why cancer cells adapt to the less efficient glycolysis for energy sources even with rich oxygen supply. We surmise that some other pathways exist to modulate Warburg effect independent of oxygen levels. To test the hypothesis that Lin28A and Lin28B regulate aerobic glycolysis independent of oxygen or HIF-1, the HIF-1α knockdown Hep3B and SK-HEP-1 cell lines were used ( Fig. 6a and Supplementary Fig. 12A ). Interestingly, under normoxic condition, Lin28A or Lin28B overexpression led to an increase in PDK1 protein in both HIF-1α knockdown and their control cells ( Fig. 6b,c and Supplementary Fig. 12B,C ). Furthermore, we found that Lin28A or Lin28B displayed similar effect in terms of enhancing glucose uptake or lactate production in HIF-1α knockdown cells compared with their control cells ( Fig. 6d,e ), suggesting that Lin28A- and Lin28B-regulated glucose metabolism via PDK1 was independent of HIF-1. Taken together, our observation established a novel mechanism by which Lin28/let-7 axis facilitates glycolytic metabolism in a way that is independent of oxygen or HIF-1 in cancer cells ( Fig. 6f ). 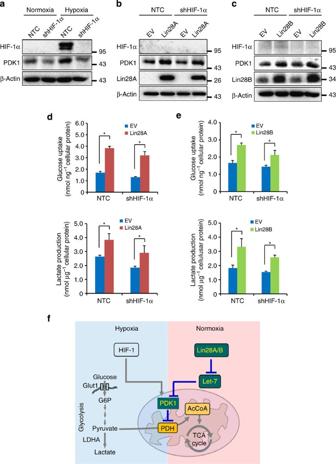Figure 6: Lin28-regulated cancer cell metabolism is HIF-1-independent. (a) Hep3B cells stably expressing NTC or shHIF-1α were incubated under normoxia or hypoxia for 4 and 48 h, respectively, followed by western blot analysing HIF-1α and PDK1. β-Actin served as loading control. (b,c) Hep3B cells stably expressing NTC or shHIF-1α were infected with viruses expressing Lin28A (b) or Lin28B (c) and cultured under normoxic condition. PDK1, HIF-1α, Lin28A and Lin28B protein levels were determined by western blot. β-Actin served as loading control. (d,e) Hep3B cells stably expressing NTC or shHIF-1α were infected with viruses expressing Lin28A (d) or Lin28B (e), followed by measurement of cellular glucose uptake and lactate production in the medium. Data were presented as mean (±s.d.).n=3 in each group. *P<0.05 as compared with indicated group (Student’st-test). (f) Summary of this study: Results in this study demonstrated that Lin28/let-7 axis regulates PDK1 in a way that is independent of oxygen or HIF-1. Together with previous studies that established PDK1 as a direct target of HIF-1, we propose that PDK1 is a master switcher of cancer cell metabolism under both aerobic and hypoxic conditions. Figure 6: Lin28-regulated cancer cell metabolism is HIF-1-independent. ( a ) Hep3B cells stably expressing NTC or shHIF-1α were incubated under normoxia or hypoxia for 4 and 48 h, respectively, followed by western blot analysing HIF-1α and PDK1. β-Actin served as loading control. ( b , c ) Hep3B cells stably expressing NTC or shHIF-1α were infected with viruses expressing Lin28A ( b ) or Lin28B ( c ) and cultured under normoxic condition. PDK1, HIF-1α, Lin28A and Lin28B protein levels were determined by western blot. β-Actin served as loading control. ( d , e ) Hep3B cells stably expressing NTC or shHIF-1α were infected with viruses expressing Lin28A ( d ) or Lin28B ( e ), followed by measurement of cellular glucose uptake and lactate production in the medium. Data were presented as mean (±s.d.). n =3 in each group. * P <0.05 as compared with indicated group (Student’s t -test). ( f ) Summary of this study: Results in this study demonstrated that Lin28/let-7 axis regulates PDK1 in a way that is independent of oxygen or HIF-1. Together with previous studies that established PDK1 as a direct target of HIF-1, we propose that PDK1 is a master switcher of cancer cell metabolism under both aerobic and hypoxic conditions. Full size image PDK1 is critical for Lin28A/B-mediated tumour proliferation Since our results have demonstrated clearly that Lin28A and Lin28B regulate aerobic glycolysis in cancer cells via PDK1, we further explored whether PDK1 is critical for Lin28A- and Lin28B-regulated cancer proliferation. First, we knocked down PDK1 in Hep3B cells stably expressing green fluorescent protein (GFP)-Lin28A or GFP-Lin28B ( Fig. 4c,d ). Cell growth analysis revealed that knockdown PDK1 diminished the promoting effect of Lin28A and Lin28B on cell proliferation ( Fig. 7a ). Xenograft experiments in nude mice demonstrated significantly enhanced tumour size and tumour mass in Hep3B cells stably overexpressing Lin28A or Lin28B compared with control group ( Fig. 7b,c and Supplementary Fig. 13A ). However, when PDK1 was knocked down, Lin28A- or Lin28B-enhanced tumour growth was obviously restrained ( Fig. 7b,c and Supplementary Fig. 13A ). Lysates from tumour tissues revealed that tumours generated from Lin28A and Lin28B overexpressing cells had higher PDK1 expression ( Fig. 7d ). Next, we overexpressed GFP-PDK1 in Hep3B cells expressing shLin28A or shLin28B. Downregulation of Lin28A or Lin28B by shRNAs markedly reduced cell growth in vitro ( Fig. 7e ) as well as tumour growth in vivo ( Fig. 7f,g and Supplementary Fig. 13B ). Forced expression of PDK1 rescued the impairment of tumour growth by shLin28A or shLin28B both in vitro and in vivo ( Fig. 7e–g and Supplementary Fig. 13B ). Western blotting of tumour tissue lysates confirmed the overexpression of PDK1 and the downregulation of Lin28A and Lin28B by their shRNAs ( Fig. 7h ). These results demonstrate that PDK1 is critical for Lin28A- and Lin28B-mediated tumour proliferation both in vitro and in vivo. Of note, shLin28 was also observed to affect growth of PDK1 overexpressing cells in vivo ( Fig. 7f,g ), possibly by inhibiting endogenous PDK1 or through other unknown mechanisms. 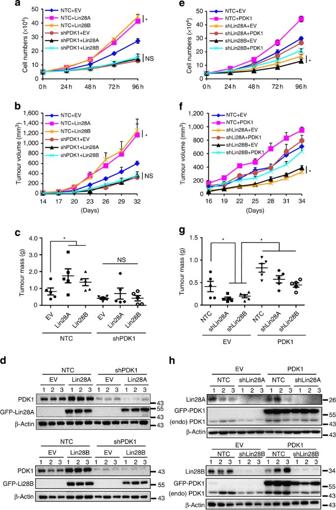Figure 7: PDK1 is critical for Lin28A/B-mediated tumour proliferation. (a) Hep3B cells stably overexpressing GFP-Lin28A or GFP-Lin28B were further infected with viruses expressing NTC or shPDK1, followed by cell growth analysis using Trypan blue staining. Data were presented as mean (±s.d.).n=3 in each group. *P<0.05 as compared with NTC+EV (empty vector) group. (Student’st-test). (b–d) Hep3B cells used in (a) were injected subcutaneously into the flanks of BALB/c nude mice (n=5 in each group). Tumour sizes were measured every 3 days using caliper (b). Tumours were extracted and tumour mass were measured at the end of experiment (c), followed by western blot determining protein levels of PDK1, Lin28A and Lin28B (d). β-Actin served as loading control. Data were presented as mean (±s.e.). *P<0.05 as compared with NTC+EV group (b) or compared with indicated group (c). NS, not significant. (Student’st-test). (e) Hep3B cells stably expressing NTC, shLin28A or shLin28B were further infected with viruses expressing GFP-PDK1, followed by cell growth analysis using Trypan blue staining. Data were presented as mean (±s.d.). *P<0.05 as compared to NTC+EV group. (Student’st-test). (f–h) Hep3B cells used in (e) were injected subcutaneously into the flanks of BALB/c nude mice (n=5 in each group). Tumour sizes were measured every 3 days using caliper (f). Tumours were extracted and tumour mass were measured at the end of experiment (g), followed by western blot determining protein levels of PDK1, Lin28A and Lin28B (h). β-Actin served as loading control. Data were presented as mean (±s.e.). *P<0.05 as compared with NTC+EV group (f) or compared with indicated group (g). (Student’st-test). Figure 7: PDK1 is critical for Lin28A/B-mediated tumour proliferation. ( a ) Hep3B cells stably overexpressing GFP-Lin28A or GFP-Lin28B were further infected with viruses expressing NTC or shPDK1, followed by cell growth analysis using Trypan blue staining. Data were presented as mean (±s.d.). n =3 in each group. * P <0.05 as compared with NTC+EV (empty vector) group. (Student’s t -test). ( b – d ) Hep3B cells used in ( a ) were injected subcutaneously into the flanks of BALB/c nude mice ( n =5 in each group). Tumour sizes were measured every 3 days using caliper ( b ). Tumours were extracted and tumour mass were measured at the end of experiment ( c ), followed by western blot determining protein levels of PDK1, Lin28A and Lin28B ( d ). β-Actin served as loading control. Data were presented as mean (±s.e.). * P <0.05 as compared with NTC+EV group ( b ) or compared with indicated group ( c ). NS, not significant. (Student’s t -test). ( e ) Hep3B cells stably expressing NTC, shLin28A or shLin28B were further infected with viruses expressing GFP-PDK1, followed by cell growth analysis using Trypan blue staining. Data were presented as mean (±s.d.). * P <0.05 as compared to NTC+EV group. (Student’s t -test). ( f – h ) Hep3B cells used in ( e ) were injected subcutaneously into the flanks of BALB/c nude mice ( n =5 in each group). Tumour sizes were measured every 3 days using caliper ( f ). Tumours were extracted and tumour mass were measured at the end of experiment ( g ), followed by western blot determining protein levels of PDK1, Lin28A and Lin28B ( h ). β-Actin served as loading control. Data were presented as mean (±s.e.). * P <0.05 as compared with NTC+EV group ( f ) or compared with indicated group ( g ). (Student’s t -test). Full size image In the present study, we demonstrated that Lin28A and Lin28B promote aerobic glycolysis in cancer cells while let-7 suppresses this process via its downstream effecter PDK1 in an oxygen- or HIF-1-independent manner. Importantly, our results further demonstrated that PDK1 expression is critical for Lin28A- and Lin28B-mediated tumour proliferation in vivo . Thus, we provided a previously unappreciated post-transcriptional regulatory mechanism to explain, at least partially, how cancer cells facilitated metabolic switch to less efficient glycolysis to promote cancer progression. Together with previous results in diabetic models [4] , [29] , ESC cells [16] , [17] and during tissue repair [18] , our data in cancer cells greatly extended the role of Lin28/let-7 axis as a master regulator of metabolism in homeostasis and diseases. Nevertheless, although Lin28/let-7 axis regulates metabolism under different conditions, the mechanisms involved could be different. In mouse diabetic models, Zhu et al. [4] demonstrated that Lin28/let-7 axis activated the PI3K-Akt pathway, which subsequently activated insulin signalling and glucose metabolism. However, in mouse ESC cells, Shyh-Chang et al. [17] reported a different mechanism used by Lin28/let-7 in regulation of threonine metabolism. Shyh-Chang et al. [18] also reported recently that Lin28A bound to and enhanced the translation of mRNAs for several metabolic enzymes, thereby increasing not only glycolysis but also OXPHOS during tissue repair. Since the PI3K-Akt-mTOR pathway is one of the most commonly activated pathways in human cancers, we first set about to determine the activation status of this pathway in cancer cells when Lin28 or let-7 expression was manipulated. Surprisingly, we only observed marginal changes of AKT or RPS6 phosphorylation, the proxy of PI3K-Akt-mTOR activation, when Lin28 expression was changed ( Supplementary Fig. 7 ). These results prompted us to seek other metabolism-related effectors regulated by Lin28 or let-7. Studies of metabolic enzymes in cell lines with altered expression of Lin28A, Lin28B and let-7g led us to the discovery of changes of PDK1, a key enzyme that is known as a regulator of cancer metabolism in tumour hypoxic microenvironment ( Figs 4a and 5a ). We further established PDK1 as a direct effecter of Lin28/let-7 axis by following evidence: first, results from gain-of-function and loss-of-function experiments of Lin28A, Lin28B and let-7g confirmed that Lin28A and Lin28B increased, whereas let-7 inhibited, PDK1 protein level in different cancer cells ( Figs 4a,b and 5a,b and Supplementary Figs 4A,F, 9A and 11A ); second, bioinformatic analysis predicted that PDK1 was a direct target of let-7g ( Fig. 5d ); third, mutagenesis experiments proved that let-7g did directly regulate PDK1 at post-transcriptional level ( Fig. 5e ); fourth, PDK1 knockdown in Lin28A/B overexpression or let-7g inhibition conditions abolished Lin28/let-7-mediated metabolism reprogramming ( Figs 4c,d and 5f ); and finally, the significantly decreased PDH activity in Hep3B stably expressing Lin28A and Lin28B suggests that TCA cycle and OXPHOS were suppressed while let-7 plays the opposite role ( Supplementary Fig. 10 ). Taken together, these results clearly demonstrated that PDK1 was responsible, at least in part, for Lin28/let-7 axis-mediated metabolic switch in cancer cells. Our discovery of PDK1 as a major effecter in Lin28/let-7-mediated glycolysis is very interesting. It is well appreciated that a central stress that cancer cells have to face during cancer development is the hypoxic microenvironment. As a common strategy for many cancers, HIF-1, a master regulator of cellular response to hypoxic stress, is activated to help adapt the situation by serials of changes to improve angiogenesis, metabolism and so on [21] . An elegant model by Kim et al . [24] described that, under hypoxic condition, HIF-1 activates PDK1, which suppresses PDH. As a result, PDK1 activation by HIF-1 will shunt pyruvate entry into TCA cycle to prevent excessive production of ROS, which is toxic to cancer cells under hypoxic condition [24] , [25] . This model illustrates elegantly how cancer cells hijack cellular metabolism for survival or growth advantages under hypoxic condition and points to the opportunity of targeting metabolism to cure cancers. As a proof of concept for cancer therapy, dichloroacetate (DCA), an inhibitor of PDK1, was used to treat tumours efficiently in mouse models [30] . Of note, PDK1 was also found to be a major effecter to regulate glycolysis in hematopoietic stem cells and to facilitate induced pluripotent stem cells induction under hypoxia conditions [31] . However, while all those results clearly demonstrated the important role PDK1 plays to switch metabolism under hypoxic condition, they could not serve to answer the long-standing mystery as why cancer cells adapt the less efficient glycolysis for energy sources even with ambient oxygen supply. Hence, it is of significant interest to demonstrate here that Lin28/let-7 axis regulates glycolysis via PDK1 under normoxia. We further determined that this regulation was independent of HIF-1, as similar regulation of metabolism by Lin28/let-7 axis was observed in HIF-1 α cell lines ( Fig. 6 and Supplementary Fig. 12 ). Significantly, our xenograft results further established that the oncogenic effects of Lin28A/B are heavily relied on PDK1 expression ( Fig. 7 and Supplementary Fig. 13 ), extending the role of PDK1 as a master regulator of cancer metabolism under different contexts of oncogenic lesion or oxygen availability. Of note, we observed elevated PDK1 mRNA expression in human HCC samples ( Supplementary Fig. 14 ), suggesting that transcriptional regulation also exists for this enzyme in HCC. However, when Lin28A or Lin28B were manipulated, we observed significant changes of PDK1 only in protein levels but not that of mRNAs ( Fig. 4a,b and Supplementary Fig. 9 ), indicating that Lin28 regulated PDK1 mainly via post-transcriptional mechanism. As cancer development is often orchestrated by alterations of numerous oncoproteins or tumour suppressors and involves various mechanisms, it stands to reason that cancer metabolism is regulated by different means under various contexts, and no pathway regulating metabolism operates alone in cancer. In this regard, previous studies established that PDK1 was transcriptionally regulated by c-Myc [32] . Early reports also established the reciprocal regulation between c-Myc, Lin28 and let-7 (refs 33 , 34 ), and we confirmed this reciprocal regulation in several cell lines ( Supplementary Fig. 15 ). These results might provide insight into upstream of Lin28/let-7 axis and place this regulatory circuit under a more global oncogenic context. Nevertheless, we observed that a regulatory effect on PDK1 expression by let-7 existed even when c-Myc expression was knocked down, suggesting that Lin28/let-7 could regulate PDK1 independent of c-Myc ( Supplementary Fig. 16 ). Interestingly, an early study reported that tumour-initiating cells [35] from primary non-small cell lung cancer were observed to express high levels of Lin28B together with glycine decarboxylase, which were required for both tumor-initiating cell (TIC) growth and tumorigenesis, albeit no direct role of Lin28B on metabolism was tested in this study [36] . Hence, our results together with others clearly established lin28/let-7 axis, intertwined with other major pathways such as c-Myc, HIF-1 and PI3K-Akt under different contexts, as a major factor in cancer metabolism. Nevertheless, our in vitro and in vivo tumour growth data also indicated that both PDK1-independent roles for Lin28A/B and Lin28A/B-independent roles for PDK1 exist for tumour progression ( Fig. 7 ), suggesting that further studies are warranted to completely elucidate the molecular mechanisms by which Lin28A and B regulates cancer metabolism and progression. It has been proposed in early studies that Lin28 is an oncofetal gene with little physiological relevance in normal adult tissues [37] , [38] , suggesting therapeutic potential of targeting this pathway for human diseases. Our results demonstrated that let-7g treatment significantly increased cancer cells’ vulnerability to glutamine deprivation under both aerobic and hypoxic condition ( Supplementary Fig. 17 ). Therefore, our findings that Lin28/let-7/PDK1 axis plays vital roles in regulating cancer metabolism and cancer proliferation are of potential significance for cancer therapy. Our results suggest a novel rationale to target PDK1 for cancer therapy in malignancies with aberrant Lin28 and let-7 expression. Cell lines and cell culture HT1080, Hep3B, HepG2, PLC, SK-HEP-1, HEK293T and HEK293 cells were all obtained from American Type Culture Collection (ATCC) and maintained in DMEM (Gibco) supplemented with 10% fetal bovine serum (FBS) and 1% penicillin–streptomycin. P493-6 and PC3 cells (from ATCC) were cultured in RPMI1640 medium supplemented with 10% FBS and 1% penicillin–streptomycin. All cells were cultured in a humidified incubator at 37 °C and 5% CO 2. To repress c-Myc expression, cells were grown in the presence of 0.1 μg ml −1 tetracycline (Sigma) for indicated periods of time. Establishment of stable cells Lentiviral plasmids pSin-EF2-LIN28A -Puro, pSin-EF2-GFP-LIN28A-Puro, pSin-EF2-LIN28B-Puro pSin-EF2-GFP-LIN28B-Puro or pSin-EF2-GFP-PDK1 were co-transfected with plasmids encoding group antigen, polymerase, envelope protein and vesicular stomatitis virus G protein into HEK293T cells using Lipofectamine 2000 (Invitrogen). Viral supernatant was collected 48 h post transfection, filtered (0.45 nm pore size) and added to Hep3B cells in the presence of 8 μg ml −1 polybrene (Sigma-Aldrich). The transduced cells were selected by 0.6 μg ml −1 puromycin or sorted by flow cytometry. shRNAs targeting Lin28A or Lin28B were commercially purchased (Sigma-Aldrich). The transduction was performed using the same procedure described above. miRNA mimics and antagomirs miRNA mimics and antagomirs were purchased from Ruibo Company (Shanghai, China). An amount of 50 nM miRNA mimics or 100 nM antagomirs were transfected into HT1080 or Hep3B cells in 60-mm dish with Lipofectamine 2000 (Invitrogen) according to the manufacturer’s instruction. RNA isolation and real-time quantitative PCR miRNAs were extracted using the mirVana miRNA isolation Kit (Ambion) from cultured cells, followed by converting to cDNA using SuperScript III Reverse Transcriptase (Invitrogen). Cellular total mRNA were extracted by Trizol (Invitrogen) followed by DNase (Ambion) treatment and cDNA synthesis using iScript cDNA synthesis kit (Bio-Rad). cDNA samples were used for real-time quantitative PCR (real time (RT)–qPCR) analysis using iQ SYBR Green Supermix and the iCycler Real-time PCR Detection System (Bio-Rad). For each primer pair, annealing temperature was optimized by gradient PCR. The fold change of target mRNA expression was calculated based on threshold cycle ( Ct ), where ΔCt=Ct target −Ct 18S and Δ(ΔCt)=ΔCt control −ΔCt indicated condition . The relative amount of gene transcripts was normalized to 18S. All primers were purchased from Invitrogen. The following primers were used in reverse transcription for let-7 family members: let-7a, 5′-GTCGTATCCAGTGCAGGGTCCGAGGTATTCGCACTGGATACGACAACTAT-3′; let-7c, 5′-GTCGTATCCAGTGCAGGGTCCGAGGTATTCGCACTGGATACGACAACCAT-3′; let-7d, 5′-GTCGTATCCAGTGCAGGGTCCGAGGTATTCGCACTGGATACGACACTATG-3′; let-7f, 5′-GTCGTATCCAGTGCAGGGTCCGAGGTATTCGCACTGGATACGACAACTAT-3′; let-7g, 5′-GTCGTATCCAGTGCAGGGTCCGAGGTATTCGCACTGGATACGACAACTGT-3′. The following primers were used for RT–qPCR for let-7 family members: let-7a, 5′-GCCGCTGAGGTAGTAGGTTGTA-3′; let-7c, 5′-GCCGCTGAGGTAGTAGGTTGTA-3′; let-7d, 5′-GCCGCAGAGGTAGTAGGTTGC-3′; let-7f, 5′-GCCGCTGAGGTAGTAGATTGAT-3′; let-7g, 5′-GCCGCTGAGGTAGTAGTTTGT-3′. The following primers were used for RT–qPCR for Lin28A, Lin28B and PDK1: Lin28A: forward: 5′-CAAAAGGAAAGAGCATGCAGAA-3′; reverse: 5′-ATGATCTAGACCTCCACAGTTGTAGC-3′; Lin28B: forward: 5′-AGCCCCTTGGATATTCCAGTC-3′; reverse: 5′-AATGTGAATTCCACTGGTTCTCCT-3′; PDK1: forward: 5′-ACCAGGACAGCCAATACAAG-3′; reverse: 5′-CCTCGGTCACTCATCTTCAC-3′. Luciferase assay PDK1-3′UTR and PDK1-3′UTR-mut were inserted into the pSI-CHECK-2 dual-luciferase reporter vector, designated as pSI-PDK1-3′UTR and pSI-PDK1-3′UTR-mut, respectively. HEK293 cells were co-transfected with either pSI-PDK1-3′UTR or pSI-PDK1-3′UTR-mut along with let-7g mimics or NTC using Lipofectamine 2000 (Invitrogen) in a 48-well plate. Luciferase activity was measured 48 h after transfection using the Dual-Luciferase Reporter Assay System (Promega). Renilla luciferase was normalized to firefly luciferase activity. Western blot Total protein was isolated from cells using RIPA buffer (50 mM Tris-HCl, pH 8.0, 150 mM NaCl, 5 mM EDTA, 0.1% SDS and 1% NP-40) supplemented with cocktail. Protein concentration was measured using the Bradford assay kit. Equal amount of proteins were loaded and separated by SDS–polyacrylamide gel electrophoresis. Antibodies for Lin28A, Lin28B, pAKT, AKT, RPS6-P, RPS6 (Cell Signaling Technology; 1:1,000), c-Myc (Santa Cruz Biotechnology; 1:1,000), PDK1 (Enzo Life Sciences; 1:1,000), HIF-1α (BD Biosciences; 1:1,000), and PGK1, LDHA, HK2, GLUT1, SDHA, PDP2, TPI-1, PDHA, MDH1, ENO1, CS, FH, IDH2 (Proteintech; 1:1,000) were used for blotting. β-Actin (Abmart; 1:5,000) served as loading control. The uncropped scans of western blots are shown in the Supplementary Fig. 18 . Measurement of lactate production The extracellular lactate was measured using the cell culture medium with lactate assay kit (BioVision) according to the manufacturer’s instruction. The values were normalized to the protein concentration. Measurement of glucose uptake Intracellular glucose was measured using cell lysates with glucose assay kit (BioVision) according to the manufacturer’s instruction. The values were normalized to the protein concentration. Measurement of cellular O 2 consumption Cells were trypsinized and suspended at 5 × 10 6 cells ml −1 in DMEM supplemented with 10% FBS. For each set of experiments, equal numbers of cells in a 0.5-ml volume were placed into the chamber of an Oxytherm unit (Strathkelvin Instrument Ltd), which uses a Clark-type microelectrode to monitor the dissolved O 2 concentration in the sealed chamber over time. The data were exported to a computerized chart recorder (Strathkelvin 782 System, Strathkelvin Instrument Ltd), which calculated the rate of O 2 consumption. The temperature was maintained at 25 °C during the measurement. Measurement of ATP production ATP levels were measured using an ATP assay kit (Celltiter-Glo Luminescent Cell Viability Assay, Promega) according to the manufacturer’s instructions. Luminescence was measured using a luminescence reader (Promega) and the values were normalized to the protein concentration. Animal studies All animal studies were conducted with approval from the Animal Research Ethics Committee of the University of Science and Technology of China. For xenograft experiments, Hep3B cells with GFP-Lin28A or GFP-Lin28B overexpression were further infected with NTC viruses or viruses expressing shRNA targeting PDK1. In a complementary assay, Hep3B cells stably expressing NTC, shLin28A or shLin28B were infected with viruses expressing empty vector or GFP-PDK1. Male BALB/c nude mice were purchased from SJA Laboratory Animal Company of China, which were randomly assigned to experimental groups. Equal numbers of the established stable cells were injected subcutaneously into nude mice. Fourteen or 16 days after injection, tumour volumes were measured every 3 days with a caliper and calculated using the equation, volume=width × depth × length × 0.52. Clinical human HCC specimens Human tissue specimens, including 17 pairs of freshly snap-frozen HCC tissues and paired normal adjacent tissues, were histopathologically diagnosed at Yat-sen University Cancer Center (Guangzhou, China). For using of these clinical materials for research purposes, prior patient’s written informed consents and approval from the Institutional Research Ethics Committee of Sun Yat-sen University Cancer Center were obtained. Total RNA was extracted from those tissues followed by real-time quantitative PCR analysis. siRNA transfection siRNA oligos targeting Lin28A and Lin28B were purchased from Ruibo Company (Shanghai, China). siRNAs targeting Lin28A are as follows: (1) 5′-GCAGTGGAGTTCACCTTTA-3′ and (2) 5′-GAAGAAATCCACAGCCCTA-3′. siRNAs targeting Lin28B are as follows: (1) 5′-GGATATTCCAGTCGATGTA-3′ and (2) 5′-GGAGATAGATGCTACAACT-3′. siRNAs were transfected into Hep3B cells by using C10511-03 riboFECT CP Transfection Kit (Ruibo) according to the manufacturer’s instruction. Twenty-four hours after transfection, Hep3B cells were re-seeded into 12-well plates, followed by cell counting with Trypan blue staining at the indicated time. Measurement of PDH activity Intracellular PDH activity was measured using cell lysates with PDH activity assay kit (BioVision) according to the manufacturer’s instruction. The values were normalized to the protein concentration. Statistical analysis The data were presented as mean±s.d. or mean±s.e. Student’s t- test was used to calculate P values. Statistical significance is displayed as * P <0.05. How to cite this article: Ma, X. et al. Lin28/let-7 axis regulates aerobic glycolysis and cancer progression via PDK1. Nat. Commun. 5:5212 doi: 10.1038/ncomms6212 (2014).